Conformational flexibility and changes underlying activation of the SUMO-specific protease SENP1 by remote substrate binding Ubiquitin-like (Ubl) modifications regulate nearly all cellular functions in eukaryotes with the largest superfamily of Ubl-specific proteases being Cys proteases. SENP1 is a model for this protease family and responsible for processing SUMO. Here using nuclear magnetic resonance relaxation measurements, chemical shift perturbation and enzyme kinetic analysis, we provide structural insights into the mechanism of substrate recognition coupled enzymatic activation within SENP1. We find that residues in the catalytic channel of SENP1, including the ‘lid’ residue Trp465, exhibit dynamics over a range of timescales, both in the presence and absence of bound substrates. The β-grasp domain of SUMO1 alone induces structural changes at ~20 Å away in the active site of SENP1, revealing the importance of this domain in activating the enzyme. These findings likely represent general properties of the mechanism of substrate recognition and processing by SENPs and other Ubl-specific proteases, and illuminate how adaptive substrate binding can allosterically enhance enzyme activity. Ubiquitin-like (Ubl) modifications play essential roles in cellular regulation in eukaryotes, and Cys proteases form the largest superfamily of Ubl-specific proteases [1] . All small Ubl modifier (SUMO)-specific proteases belong to this family, as do at least four types of de-ubiquitination enzymes (DUBs)—ubiquitin-specific proteases (USP), ovarian tumour proteases, Machado–Josephin domain proteases and the ubiquitin C-terminal hydrolases [2] . Ubls, such as ubiquitin and SUMO, are first synthesized as precursor proteins that are cleaved by Ubl-specific proteases to expose their C-terminal Gly–Gly motif. After being cleaved, a Ubl is conjugated to other cellular proteins through the functions of three enzymes—generally known as E1, E2 and E3 (refs 3 , 4 , 5 ). Ubl-specific proteases also remove Ubls from modified proteins when regulating these dynamic modifications. SUMO-specific proteases include SENP1, 2, 3, 5, 6 and 7, and USPL1 (refs 6 , 7 ). These Cys proteases have similar biochemical mechanisms, and available crystal structures have revealed common structural features at their catalytic centres. These previous studies have also inspired some general questions regarding their catalytic mechanisms. First, the catalytic Cys residues are located within the closed catalytic channels for binding the C-termini of Ubls ( Fig. 1a , Supplementary Fig. 1 ) [8] , [9] , [10] , [11] , [12] , [13] , [14] , [15] . In all SENPs, an aromatic side chain, such as that of Trp or Phe, forms the channel ‘lid’ (Fig. 1a , Supplementary Fig. 1 ). It remains unclear how substrates bind into the closed catalytic channels to reach the catalytic Cys. Second, the catalytic residues undergo conformational changes when these proteases form complexes with their substrates [12] , [13] , [16] , [17] . The mechanisms for rearranging the catalytic residues are not well-understood. 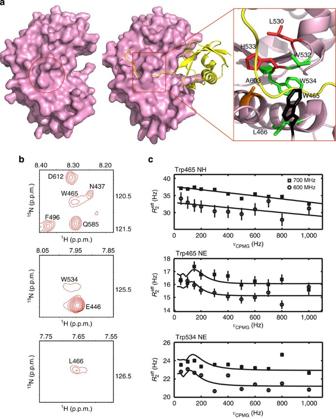Figure 1: Characterization of the conformational dynamics of apo-SENP1 (C603S). (a) The closed catalytic channel of SENP1. SENP1 is shown as surface representation and the closed catalytic channel in apo-SENP1 (pdbid: 2IYC) is indicated with a circle (left panel). SUMO1 is shown in ribbon diagram (middle and right panels, pdbid:2IY1). A zoom-in view of the catalytic channel (right panel) is shown with side chains that are labelled with their residue numbers and coloured according to the timescale of their conformational dynamics. Red, microsecond dynamics detected by HzNzR1ρ only; green, micro–millisecond dynamics detected by CPMG only; and black, pico–millisecond dynamics detected by1H–15N NOE, HzNzR1ρ and CPMG. (b) Representative broadened backbone NH resonances of residues Trp465, Trp534 and Leu466 that are at or near the catalytic channel from the1H–15N HSQC spectrum of apo-SENP1. (c) Representative CPMG-relaxation dispersion profiles for the resonances of residues at the catalytic channel, measured by 600 (circle) and 700 (square) MHz NMR instruments. The error bars were obtained from duplicated measurements (see Methods section). Figure 1: Characterization of the conformational dynamics of apo-SENP1 (C603S). ( a ) The closed catalytic channel of SENP1. SENP1 is shown as surface representation and the closed catalytic channel in apo-SENP1 (pdbid: 2IYC) is indicated with a circle (left panel). SUMO1 is shown in ribbon diagram (middle and right panels, pdbid:2IY1). A zoom-in view of the catalytic channel (right panel) is shown with side chains that are labelled with their residue numbers and coloured according to the timescale of their conformational dynamics. Red, microsecond dynamics detected by H z N z R 1 ρ only; green, micro–millisecond dynamics detected by CPMG only; and black, pico–millisecond dynamics detected by 1 H– 15 N NOE, H z N z R 1 ρ and CPMG. ( b ) Representative broadened backbone NH resonances of residues Trp465, Trp534 and Leu466 that are at or near the catalytic channel from the 1 H– 15 N HSQC spectrum of apo-SENP1. ( c ) Representative CPMG-relaxation dispersion profiles for the resonances of residues at the catalytic channel, measured by 600 (circle) and 700 (square) MHz NMR instruments. The error bars were obtained from duplicated measurements (see Methods section). Full size image SENP1 is a model system for the Ubl-specific proteases in the Cys protease superfamily because it shares the same biochemical mechanism and its catalytic Cys is similarly buried as those of other Ubl-specific proteases ( Fig. 1a , Supplementary Fig. 1 ) [10] , [11] , [12] , [13] , [14] . In addition, SENP1 is an essential gene and is a potential target for developing new therapeutic agents for cancer. SENP1 plays a key role in tumour angiogenesis, because it regulates the stability of hypoxia-inducible factor 1α, which is a key player in the formation of new blood vessels to support tumour growth [18] , [19] . SENP1 is also highly expressed in human prostate cancer specimens and regulates androgen receptor activities [20] , [21] , [22] . Similarly, many Ubl-specific proteases are targets for developing therapies for life-threatening diseases such as cancer, neurodegenerative disorders and infectious diseases [20] , [21] , [23] , [24] , [25] . Despite the availability of many crystal structures, it has been challenging to develop competitive inhibitors that target the catalytic channel [26] , suggesting that a better understanding of these enzymes and their interactions with substrates is necessary. To address some of the outstanding questions for this class of enzymes, we performed nuclear magnetic resonance (NMR) studies on SENP1 in combination with enzyme kinetic analysis. Although crystal structures show the catalytic channel of SENP1 to be closed, we find that these residues exhibit extensive motions that likely reflect open–closed dynamics; moreover, these dynamics persist in the presence of bound substrate. In addition, we have found that the distally bound β-grasp domain of SUMO1 induces realignment of the catalytic residues that enhance the enzyme activity. Similar enhancement has also been observed for a DUB, USP5. We suggest that the mode of substrate recognition and binding we observed for SENP1 may be shared by other de-Ubl enzymes. Conformational dynamics of the catalytic channel Although crystal structures show that the catalytic Cys residue of SENP1 is located within closed catalytic channel ( Fig. 1a ) [13] , [14] , extensive conformational flexibility on the micro–millisecond timescale is apparent for residues at the catalytic channel based on their severely broadened resonances in the 1 H– 15 N HSQC spectra ( Fig. 1b ). These spectra and other data were obtained with the catalytically inactive C603S mutant of SENP1 catalytic domain to compare the free enzyme with enzyme–substrate complexes as discussed below. Similar flexibility is expected for the wild-type (WT) SENP1, because severe line broadening was observed for the amide resonances of the residues at the catalytic channel, including Trp534 ( Supplementary Fig. 2 ) and residues 464–466, whose amide resonances were too broad to be observed in the 1 H– 15 N HSQC spectrum. These dynamics were characterized by measuring the 15 N R 1 , R 2 , 1 H– 15 N nuclear Overhauser effect (NOE) and H z N z R 1 ρ relaxation rates, as well as 15 N and 13 C-methyl Carr–Purcell–Meiboom–Gill (CPMG)-transverse relaxation dispersion for the C603S mutant ( Supplementary Tables 1–4 and Supplementary Fig. 3 ). These measurements were designed to provide quantitative information of dynamics over a wide range of timescales. 1 H– 15 N NOE and 15 N R 1 rates are sensitive to motions on the pico–nanosecond timescale that reflects the conformational entropy of the system, while R ex of H z N z R 1 ρ detects dynamics on the microsecond timescale [27] . CPMG-relaxation dispersion provides insights into conformational dynamics on a timescale (micro–millisecond) slower than what can be detected by R 1 ρ. Protein dynamics in the micro–millisecond timescale are associated with molecular recognition and enzyme catalysis. The slower the dynamics, the higher the energy barrier of the changes between the different conformational states according to thermal dynamic principles. Relaxation measurements on free SENP1 reveal that the catalytic channel of SENP1 undergoes extensive dynamics over a wide range of timescales. The catalytic channel lid Trp465 undergoes motions over the widest timescales, from pico to millisecond, among detectable resonances of residues at the catalytic channel, also consistent with its broadened amide resonances ( Fig. 1b ). Fast motions in the pico–nanosecond timescale regime for Trp465 are indicated by 1 H– 15 N NOE values ( Supplementary Table 3 ) less than the theoretical maximum (~0.83 at 600 MHz spectrometer frequency) observed for Trp465 (0.66 for the backbone N and 0.57 for the side chain Nε, Supplementary Table 3 ). 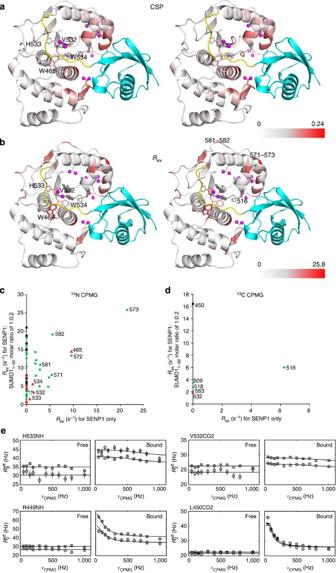Figure 3: Allosteric effect of SUMO11–92on the catalytic channel as detected by CSP and CPMG-relaxation dispersion. (a) Stereo view of SENP1 structure coloured according to CSP (calculated as) caused by formation of the complex with SUMO11–92. The gradient from white to red corresponds to the CSP (from small to large) of backbone NH groups. Above average CSP (0.05 p.p.m.) of the methyl groups are indicated by magenta ball and stick figures. (b) Stereo view of SENP1 structure coloured according to theRexvalues extracted from the fitted CPMG-relaxation dispersion profiles of the SENP1:SUMO11–92complex at molar ratio of 1:0.2. The gradient from white to red corresponds to theRex(from small to large). Substantial methyl CPMG-relaxation dispersion is indicated by magenta ball and stick figures. In bothaandb, key residues at the catalytic channel are shown with their side chains and labelled. SUMO11–92is shown in cyan, and the C-terminal segment in SUMO1-FL is shown in yellow on the crystal structure of the complex between SUMO1-FL and SENP1 (PDB: 2IY1). (c,d) Comparison ofRexextracted from CPMG-relaxation dispersion between free SENP1 and SENP1 in complex with a 0.2 molar equivalence of SUMO11–92detected by15N-CPMG dispersion (c) and13C-methyl-CPMG dispersion (d). Residues at the direct binding surface for the β-grasp domain (defined as the buried surface by SUMO11–92as provided by the Interface Residues script,http://www.pymolwiki.org/index.php/InterfaceResidues, of the software pymol) are indicated in black, at the catalytic centre in red (defined as contacting the residues 96–98 of SUMO1-FL), and at neither the catalytic centre nor the direct binding surface in green. (e) Representative CPMG dispersion profiles of the resonances of SENP1 residues at 600 (circle) and 700 (square) MHz NMR instruments when free and partially bound to SUMO11–92. Error bars were obtained from duplicated measurements. In addition, significant motions in the microsecond timescale were detected by H z N z R 1 ρ measurements ( Supplementary Table 4 ) [27] . 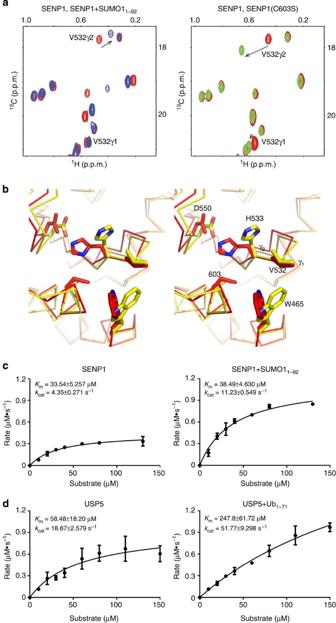Figure 4: The critical role of the β-grasp domain of SUMO1 on binding and activity enhancement of SENP1. (a) Left panel, overlap of the1H–13C-methyl TROSY spectra of SENP1 (red), and SENP1 in complex with SUMO11–92complex (blue). Right panel, overlay of the spectra of wild-type SENP1 (green) and SENP1 (C603S) (red). Stereo-specific assignments of the Val532 methyl groups are indicated. (b) Stereo view of representative SENP1 crystal structures showing Val532 and surrounding residues for relating structural changes to the observed chemical shift changes in the methyl groups of Val532 shown ina. The Val532 γ2-methyl group faces the His533 aromatic ring while the γ1-methyl group is pointing away. The PDB IDs for the structures are: red-2IYC (apo-state) and yellow-2IY0 (complex state). (c) Steady-state kinetic measurements for SENP1, free (left panel) and when saturated with SUMO11–92(right), using DUB-Glo as a substrate. The fitted kinetic parameters are shown with the corresponding data. (d) Steady-state kinetic measurements for USP5, free (left panel) and when saturated with ubiquitin1–71(right), using DUB-Glo as a substrate. The fitted kinetic parameters are shown with the corresponding data. Forcandd, error bars were obtained from triplicated measurements. Furthermore, 15 N-CPMG dispersions were observed for both Trp465 N and Nε groups by 600 and 700 MHz NMR instruments, indicating dynamics in the micro–millisecond timescale ( Fig. 1c ). The CPMG dispersion profiles of the Trp465 backbone and side chain did not plateau at the highest CPMG field strength ( Fig. 1c ), consistent with the motions detected for this residue by H z N z R 1 ρ. Trp534 at the bottom of the catalytic channel undergoes micro–millisecond timescale dynamics, as indicated by 15 N-CPMG dispersion for Nε by the 600 and 700 MHz NMR instruments ( Fig 1a,c ). His533, which is involved in catalysis, and Leu530, which is near His533, undergo microsecond timescale motions as indicated by the large R ex values obtained from the H z N z R 1 ρ measurements ( Fig. 1a , Supplementary Table 4 ). The fast motions of His533 suggest that it is susceptible to conformational changes. SENP1 interaction with substrates The substrate SUMO1 consists of a β-grasp domain that encompasses residues 20–92 and a flexible C terminus that begins with residue 93 in the SUMO1 precursor (referred to as SUMO1-FL, residues 1–101) or in mature SUMO1 (referred to as SUMO-GG, residues 1–97) that is the product of SENP1 cleavage. Both the β-grasp domain and the unstructured C terminus interact with SENPs in the crystal structures of their complexes with SUMO precursors or conjugated substrates [10] , [11] , [12] , [13] , [14] . We compared SENP1 interactions with SUMO1-FL, SUMO1-GG, SUMO1 1–92 (containing residues 1–92, with C terminus truncated) or peptides corresponding to the C terminus of SUMO1. Each of these SUMO1 constructs was titrated into 15 N or 13 C-methyl-labelled SENP1, and NMR chemical shift perturbation (CSP) was monitored in a series of two-dimensional 1 H– 15 N HSQC or 1 H– 13 C HMQC correlation spectra ( Fig. 2a–d,f,g and Supplementary Fig. 4 ). The exchange rates between free SENP1 and SENP1 in complex with SUMO1-FL or SUMO1-GG were mostly slow to intermediate, relative to the NMR chemical shift timescale, and both SUMO-GG and SUMO-FL produced similar CSP ( Fig. 2b ). Upon titration with SUMO1 1–92 , the resonances of some residues (that is, R449; Fig. 2c and Supplementary Fig. 4 ) showed similarly slow exchange between free and bound states and similar CSP as that observed for binding of SUMO1-FL or SUMO1-GG. The resonances of some other residues (that is, T451 and Q507; Fig. 2c and Supplementary Fig. 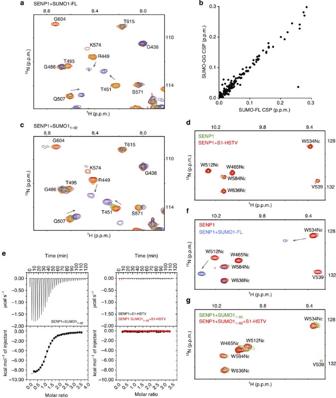4 ) showed fast exchange between the free and bound states but with similar CSP trends. These data suggest that the β-grasp domain of SUMO1 interacts with SENP1 in a manner similar to that in the context of SUMO1-FL. Figure 2: Characterization of the binding of SUMO1 constructs to SENP1. (a) Representative region of the superimposed1H–15N HSQC spectra for monitoring the titration of SENP1 with SUMO1-FL. Spectra are coloured as a rainbow from red to violet, corresponding to increasing SENP1:SUMO1 molar ratios (1:0, 1:0.2, 1:0.4, 1:0.6, 1:0.8, 1:1.07 and 1:1.39). Arrows indicate the direction of CSP. (b) Correlation of CSP of SENP1 upon binding SUMO1-GG and SUMO1-FL at a SENP1:SUMO1 molar ratio of 1:1.39. (c) The same region as shown inabut of the superimposed1H–15N HSQC spectra monitoring the titration of SENP1 with SUMO11–92.(d) Overlay of the1H–15N HSQC spectra of SENP1, free (green) and in the presence of a 2.4-fold higher concentration of the S1-HSTV peptide (red). (e) ITC profiles of SENP1 titration with SUMO11–92(left), or the S1-HSTV peptide (right, black) that is superimposed onto the profile of S1-HSTV titration into the SENP1–SUMO11–92complex (right, red). (f) Overlay of a region of the1H–15N HSQC spectra showing the resonances of Trp side chains of SENP1 free (red) and in complex with SUMO1-FL (blue). (g) Overlay of the same region of the1H–15N HSQC spectra as that indandfof the SENP1–SUMO11–92complex (green), and that in the presence of a 2.7-fold higher concentration of S1-HSTV (red). Figure 2: Characterization of the binding of SUMO1 constructs to SENP1. ( a ) Representative region of the superimposed 1 H– 15 N HSQC spectra for monitoring the titration of SENP1 with SUMO1-FL. Spectra are coloured as a rainbow from red to violet, corresponding to increasing SENP1:SUMO1 molar ratios (1:0, 1:0.2, 1:0.4, 1:0.6, 1:0.8, 1:1.07 and 1:1.39). Arrows indicate the direction of CSP. ( b ) Correlation of CSP of SENP1 upon binding SUMO1-GG and SUMO1-FL at a SENP1:SUMO1 molar ratio of 1:1.39. ( c ) The same region as shown in a but of the superimposed 1 H– 15 N HSQC spectra monitoring the titration of SENP1 with SUMO1 1–92. ( d ) Overlay of the 1 H– 15 N HSQC spectra of SENP1, free (green) and in the presence of a 2.4-fold higher concentration of the S1-HSTV peptide (red). ( e ) ITC profiles of SENP1 titration with SUMO1 1–92 (left), or the S1-HSTV peptide (right, black) that is superimposed onto the profile of S1-HSTV titration into the SENP1–SUMO1 1–92 complex (right, red). ( f ) Overlay of a region of the 1 H– 15 N HSQC spectra showing the resonances of Trp side chains of SENP1 free (red) and in complex with SUMO1-FL (blue). ( g ) Overlay of the same region of the 1 H– 15 N HSQC spectra as that in d and f of the SENP1–SUMO1 1–92 complex (green), and that in the presence of a 2.7-fold higher concentration of S1-HSTV (red). Full size image In contrast, the peptides corresponding to the C terminus of SUMO1, S1-HSTV (residues 93–101, sequence of EQTGGHSTV) or S1-GG (residues 93–97 of SUMO1, sequence of EQTGG), did not produce CSP on SENP1 resonances upon titration into SENP1 ( Fig. 2d ). NMR CSP is the most sensitive method to detect weak interactions. This result indicates that the C-terminal segment of the substrate has a considerably low intrinsic affinity for the enzyme. Isothermal titration calorimetry (ITC) measurements confirmed this observation. Binding of SUMO1 1–92 to SENP1 resulted in significant heat release ( K d of 3.52±0.081 μM, Δ H of −9.3±0.14 kcal mol −1 and Δ S of −6.3 cal mol −1 K −1 ), but the S1-GG or S1-HSTV peptides did not result in significant heat exchange, as shown by the representative ITC profile of S1-HSTV binding ( Fig. 2e ). Taken together, these data suggest that the β-grasp domain of SUMO1 is the main contributor to the binding affinity to SENP1, but the C-terminal region is not. Although the C-terminal region of SUMO1 did not show detectable interaction with SENP1 by itself, NMR data indicates that this region does interact, weakly and in a dynamic manner, with SENP1 in the context of the full-length substrate. The interaction of the C-terminal region was indicated by significant chemical shift changes of Trp534 Nε, a residue forming the bottom of the substrate binding channel at the catalytic centre ( Fig. 2f,g ). The observed interaction, in contrast to the isolated S1-HSTV peptide, is unlikely due to an allosteric effect of the β-grasp domain because SUMO1 1–92 did not significantly enhance the binding of S1-GG or S1-HSTV peptides ( Fig. 2e,g ). Trp512 is located at the β-grasp domain-binding surface on SENP1, and significant chemical shift change of Trp512 Nε is observed upon binding SUMO1-FL as expected. The broadened line-width at Trp534 Nε resonance and the complete loss of Trp465 Nε resonance in the complex with SUMO1-FL in contrast to the strong resonance of Trp512 Nε ( Fig. 2f ), in combination with the intrinsic low affinity of the SUMO C terminus for SENP1, suggest that the C-terminal region swayed between bound and unbound states while the β-grasp domain was bound. In addition, the different line-broadening effects on the Trp465 and Trp534 Nε resonances ( Fig. 2f ), which form the top and bottom of the substrate binding channel, respectively ( Fig. 1a ), indicate that Trp465 continues to undergo conformational exchange in the complex, possibly open–close dynamics, and not simply the closed conformation seen in SUMO-bound SENP1 crystal structures [12] , [13] , [14] , [28] . Effects of the SUMO1 β-grasp domain on SENP1 We mapped the CSP of SENP1 induced by binding SUMO1 1–92 onto the crystal structure of SENP1 (C603A) in complex with SUMO1-FL (PDB: 2IY1) ( Fig. 3a ). This revealed that substantial CSP are not localized to the direct interaction surface on SENP1 ( Fig. 3a and Supplementary Figs 4 and 5 ), but propagated to residues at the catalytic channel and beyond, such as Trp465-Asp468 and Leu530, Trp534, His533 and Ser603. In addition, we saw CSP of methyl groups that are not located at the direct contact surface for binding the β-grasp domain, indicating that the allosteric effect was propagated from the direct contact surface through the hydrophobic core ( Fig. 3a ). The CSPs at these regions suggest that the interaction with the β-grasp-fold domain of SUMO1 induced a structural allosteric effect that included the catalytic channel. Figure 3: Allosteric effect of SUMO1 1–92 on the catalytic channel as detected by CSP and CPMG-relaxation dispersion. ( a ) Stereo view of SENP1 structure coloured according to CSP (calculated as ) caused by formation of the complex with SUMO1 1–92 . The gradient from white to red corresponds to the CSP (from small to large) of backbone NH groups. Above average CSP (0.05 p.p.m.) of the methyl groups are indicated by magenta ball and stick figures. ( b ) Stereo view of SENP1 structure coloured according to the R ex values extracted from the fitted CPMG-relaxation dispersion profiles of the SENP1:SUMO1 1–92 complex at molar ratio of 1:0.2. The gradient from white to red corresponds to the R ex (from small to large). Substantial methyl CPMG-relaxation dispersion is indicated by magenta ball and stick figures. In both a and b , key residues at the catalytic channel are shown with their side chains and labelled. SUMO1 1–92 is shown in cyan, and the C-terminal segment in SUMO1-FL is shown in yellow on the crystal structure of the complex between SUMO1-FL and SENP1 (PDB: 2IY1). ( c , d ) Comparison of R ex extracted from CPMG-relaxation dispersion between free SENP1 and SENP1 in complex with a 0.2 molar equivalence of SUMO1 1–92 detected by 15 N-CPMG dispersion ( c ) and 13 C-methyl-CPMG dispersion ( d ). Residues at the direct binding surface for the β-grasp domain (defined as the buried surface by SUMO1 1–92 as provided by the Interface Residues script, http://www.pymolwiki.org/index.php/InterfaceResidues , of the software pymol) are indicated in black, at the catalytic centre in red (defined as contacting the residues 96–98 of SUMO1-FL), and at neither the catalytic centre nor the direct binding surface in green. ( e ) Representative CPMG dispersion profiles of the resonances of SENP1 residues at 600 (circle) and 700 (square) MHz NMR instruments when free and partially bound to SUMO1 1–92 . Error bars were obtained from duplicated measurements. Full size image To confirm the allosteric effect from binding SUMO1 1–92 , we measured 15 N and 13 C-methyl-CPMG transverse relaxation dispersion for the partially SUMO1 1–92 -bound complex [29] , [30] . SUMO1 1–92 -induced relaxation dispersion was measured at 20% SUMO1 1–92 occupancy, when the SENP1 resonances were not too broad to be measured accurately while significant relaxation dispersion could be observed. The partially bound state enhances CPMG-relaxation dispersion and thus facilitates the observation of allosteric effect by SUMO1 1–92 . As expected, the resonances of most residues at the direct binding interface of SUMO1 1–92 showed substantial CPMG dispersion, consistent with exchange between the free and the β-grasp domain-bound states occurring on the micro–millisecond timescale ( Fig. 3b–e ). The resonances of many residues that were not located at the direct binding surface, including the catalytic His533 and Val532, whose resonances only showed CPMG dispersion in the partially bound state ( Fig. 3e ), indicated a change of conformational states induced by the distally bound β-grasp domain. An area that showed significant R ex from CPMG dispersion measurements that were independent of complex formation contained the methyl group of Val516 and the backbone NH groups of residues 571–573 and 581–582 ( Fig. 3b–d ). This area is not located at the direct binding surface for the β-grasp-fold domain, but may contribute to the allosteric effect that propagates from the β-grasp binding surface to the catalytic channel. Effect of the β-grasp domain on catalysis of SENP1 1 H-chemical shifts are sensitive to non-covalent interactions. Intriguingly, the two closely positioned methyl groups of Val532 showed significantly different CSPs upon binding SUMO1 1–92 ; the γ 2 -methyl 1 H of Val532 displayed an unusually large 1 H-CSP (~0.1 p.p.m.) but the γ 1 -methyl group showed a minimal 1 H-CSP ( Fig. 4a , left panel). The selective large CSP at only the γ 2 -methyl group is unlikely to be due to structural changes at Val532. The χ 1 rotomeric distribution of Val532 in SENP1, both in the free and bound states, is estimated to be 90% gauche − state and 10% gauche + state, based on the 13 C-chemical shifts [28] . This is consistent with published SENP1 crystal structures, in which Val532 was in the gauche − state [12] , [14] . Therefore, the large 1 H-CSP likely reflects structural changes of nearby residues. An aromatic ring current effect is the most likely contributor to 1 H-CSP through non-covalent interactions. Two aromatic residues, His533 and Trp465, are adjacent to Val532. The programme SHIFTX2 (ref. 31 ) was used to analyze the effect of the distance dependence of the aromatic ring current effect of His533 and Trp465 using available crystals structures to define possible structural changes. Changes in the Trp465 side chain position were expected to cause similarly large 1 H-CSP on both Val532 methyl groups because of their similar proximities to the Trp aromatic ring ( Fig. 4b ), but inconsistent with the observed 1 H-CSP ( Fig. 4a ). However, changes in the His533 position had a much larger effect on 1 H-CSP of the γ 2 -methyl than the γ 1 -methyl of Val532, a pattern that agreed with the NMR data ( Fig. 4a , left panel) and was consistent with the γ 2 -methyl facing His533 while the γ 1 -methyl was not ( Fig. 4b ). Therefore, the observed 1 H-CSP at Val532 methyl ( Fig. 4a ) likely indicates a change in the His533 position from the free state (red structure, Fig. 4b ) towards that represented by the complex state with a substrate (yellow structure, Fig. 4b ). Further support that the γ 2 -methyl of Val532 is sensitive to changes in the catalytic residues came from substituting Cys603 with Ser, which also caused a much larger 1 H-CSP at the γ 2 -methyl than at the γ 1 -methyl ( Fig. 4a , right panel). The His533 aromatic ring is hydrogen-bonded to Cys603 through a water molecule [32] , [33] , and thus it is conceivable that Cys to Ser substitution, which results in a change of O to S, would alter the hydrogen bound with the His533 aromatic ring that caused a shift in His533 position that corresponds to a larger 1 H-CSP on the γ 2 -methyl than γ 1 -methyl. The His533 conformational change is likely enabled by its intrinsic flexibility, as indicated by its having one of the largest R ex, ρ (N ξ ) values (4.2±0.2 s −1 ) ( Fig. 1a ). In addition, His533 only showed significant CPMG dispersion when partially bound by SUMO1 1–92 , supporting a conformational change at this site induced by the binding of the β-grasp domain ( Fig. 3b,c,e ). Furthermore, the resonances of residues surrounding His533, that is, Ser603 and Gly604, also displayed CSP and CPMG dispersion when partially bound with SUMO1 1–92 ( Fig. 3a,b ), which was consistent with the realignment of the catalytic residues. Figure 4: The critical role of the β-grasp domain of SUMO1 on binding and activity enhancement of SENP1. ( a ) Left panel, overlap of the 1 H– 13 C-methyl TROSY spectra of SENP1 (red), and SENP1 in complex with SUMO1 1–92 complex (blue). Right panel, overlay of the spectra of wild-type SENP1 (green) and SENP1 (C603S) (red). Stereo-specific assignments of the Val532 methyl groups are indicated. ( b ) Stereo view of representative SENP1 crystal structures showing Val532 and surrounding residues for relating structural changes to the observed chemical shift changes in the methyl groups of Val532 shown in a . The Val532 γ 2 -methyl group faces the His533 aromatic ring while the γ 1 -methyl group is pointing away. The PDB IDs for the structures are: red-2IYC (apo-state) and yellow-2IY0 (complex state). ( c ) Steady-state kinetic measurements for SENP1, free (left panel) and when saturated with SUMO1 1–92 (right), using DUB-Glo as a substrate. The fitted kinetic parameters are shown with the corresponding data. ( d ) Steady-state kinetic measurements for USP5, free (left panel) and when saturated with ubiquitin 1–71 (right), using DUB-Glo as a substrate. The fitted kinetic parameters are shown with the corresponding data. For c and d , error bars were obtained from triplicated measurements. Full size image Based on the structural changes observed at the catalytic residues we hypothesized that the catalytic activity ( k cat ) of SENPs and possibly some DUBs would be affected upon binding the β-grasp-fold domains of their respective Ubls. To test this, we conducted steady-state enzymatic kinetic analysis of SENP1 and SENP1 that was saturated with SUMO1 1–92 , using a bioluminescent-based assay and DUB-Glo (Promega) as a substrate ( Fig. 4c ). When saturated with SUMO1 1–92 , SENP1 reproducibly had a higher apparent k cat value than did free SENP1; no significant changes in the apparent K m were seen. The lack of change in the apparent K m is consistent with the similarly small CSP and heat release generated by the S1-GG or S1-HSTV peptides on SENP1 and SENP1 in complex with SUMO1 1–92 ( Fig. 2d,e,g ). Saturation of a DUB, USP5, with the β-grasp domain of ubiquitin also enhanced the k cat ( Fig. 4d ). Unlike SENP1, Usp5 displayed significant changes in the apparent K m . This result also suggests an allosteric effect at the catalytic channel from binding the β-grasp domain of ubiquitin. Because the β-grasp domain of ubiquitin is expected to be responsible for the majority of the binding affinity, the increase in the K m with DUB-Glo could be insignificant in the context of the full-length substrates that contains the β-grasp domain of ubiquitin. Taken together, our findings suggest that conformational changes induced by the β-grasp domain optimize the catalytic residues for catalysis. The data obtained in this study indicates that residues at the catalytic channel of SENP1 undergo motions over a wide range of timescales, both free and in complex with a substrate. Among residues in the catalytic channel, the dynamics of the ‘lid’ residue, Trp465, were detected over the widest timescale from pico to millisecond, indicating its extensive flexibility. Therefore the catalytic channel undergoes extensive motions that allow substrates to bind into the seemingly closed channel ( Fig. 1 ). This finding is unlikely affected by the C603S mutation, because the WT SENP1 also has weak intrinsic affinity for the C-terminal segment of SUMO1 that is not affected by binding SUMO1 1–92 ( Supplementary Figs 6 and 7 ). Trp465 undergoes extensive motions with and without interacting with SUMO-FL ( Fig. 1 and Fig. 2f ). The β-grasp domain more stably interacts with SENP1 than with the C-terminal region of SUMO1-FL, which appears to sway between bound and unbound states, while the β-grasp domain bound to SENP1 ( Figs 2f and 5 ). DUB-Glo, a pentapeptide substrate, can be cleaved by several Ubl-specific proteases in the Cys protease superfamily, even though its sequence is derived from the C terminus of ubiquitin, which is different from the sequences of the C-terminal regions of other Ubls [34] . Therefore, the lack of specificity of the Ubl-specific proteases to peptide substrates, such as DUB-Glo, suggests that the conformational flexibility at the catalytic channel, as we found for SENP1, likely represents a general property of the Ubl-specific proteases in the Cys protease superfamily. 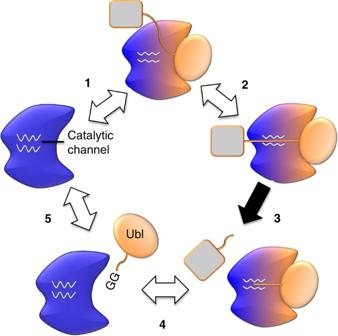Figure 5: Schematic illustration of the dynamics at the catalytic channel and the allosteric effect of the β-grasp domain. In clockwise order,1represents the catalytic channel undergoing conformational transitions,2indicates how substrate binding allosterically activates the enzyme,3indicates catalysis, and4and5indicate regeneration of the enzyme. The colour changes of a Ubl-specific protease represent allosteric effects due to binding of the β-grasp domain. Figure 5: Schematic illustration of the dynamics at the catalytic channel and the allosteric effect of the β-grasp domain. In clockwise order, 1 represents the catalytic channel undergoing conformational transitions, 2 indicates how substrate binding allosterically activates the enzyme, 3 indicates catalysis, and 4 and 5 indicate regeneration of the enzyme. The colour changes of a Ubl-specific protease represent allosteric effects due to binding of the β-grasp domain. Full size image NMR data suggest that the binding of the β-grasp domain of SUMO1 induces a structural change of the catalytic residues ( Figs 3 and 4 ). The structural changes induced by the β-grasp domain, as indicated by the selective 1 H-CSP of the γ 2 -methyl of Val532, correspond to enhanced enzymatic turnover rate of SENP1 ( Figs 4 and 5 ). Previous biochemical data indicates that our conclusion is application to all SENPs [35] , [36] . This allosteric effect from the β-grasp domain that alters the catalytic residues likely occurs in some other Ubl-specific proteases that belong to the Cys protease superfamily, as suggested by the enhanced catalysis of USP5 by the β-grasp domain of ubiquitin ( Fig. 4d ). These de-conjugation enzymes likely have high affinity for the β-grasp domain of their corresponding Ubls, such as SENPs and USP5. Our finding suggests that the previous finding that ubiquitin (not C-terminal truncated) enhances the activity of USP5 (ref. 37 ) is due to the binding of the β-grasp domain of ubiquitin. The β-grasp domain-binding surface, not only is critical to substrate binding affinity, but also responsible for enhanced activity of the Ubl-specific protease. Therefore, targeting this allosteric site in Ubl-specific proteases could be more successful in producing specific inhibitors. The role of protein–protein interactions in cellular signalling and the formation of biologically functional complexes is well appreciated. However, many proteins are also substrates for enzymes, such as those catalyzing conjugation and de-conjugation of Ubl modifications. The findings described here illustrate how a macromolecular substrate allosterically enhances the activity of its enzyme. Sample preparation His-tagged unlabelled or 15 N/ 13 C-labelled WT or C603S SENP1 catalytic domain, and unlabelled Ubl β-grasp domains, SUMO1 1–92 (deleting EQTGG) and Ubiquitin 1–71 (deleting RLRGG) were expressed and purified as described previously [34] . To overexpress selectively methyl-labelled SENP1, E. coli BL21 (DE3) cells harbouring the SENP1 plasmid were transferred into 250 ml of M9 media at 100% D2O that contained 0.25 g 15 NH 4 Cl, 1 g D 7 -glucose and sodium salts of 60 mg [methyl- 13 C; 3,3- D 2 ]-alpha-ketobutyric and 60 mg [3-methyl-13C; 3,4,4,4- D ]-alpha-ketoisovaleric acid. The cells were grown for 1 h at 37 °C prior to induction with 1 mM isopropyl β- D -1-thiogalactopyranoside for 24 h at 15 °C. All NMR isotopes were obtained from Cambridge Isotope Laboratories. The His-tagged proteins were isolated from cell lysate by using Ni-NTA (Qiagen) chromatography. The de-ubiquitin enzyme USP5 was purchased from Boston Biochem and the SUMO1 C terminus peptides, S1-HSTV (EQTGGHSTV) and S1-GG (EQTGG), were purchased from Peptide 2.0 Inc. The peptides were dissolved in D 6 -dimethyl sulfoxide (DMSO) to 20–30 mM, and their concentrations were calibrated by 1D 1 H NMR using the standard 4, 4-dimethyl-4-silapentane-1-sulphonic acid. In each experiment, <1% DMSO was introduced upon addition of the peptide and the equivalent amount of DMSO was added to record the reference spectra. NMR titration Protein samples were prepared at 0.25 mM in a buffer containing 20 mM sodium phosphate, pH 6.8, 5 mM DTT, 0.02% NaN 3 and 10% D 2 O. Chemical shift assignments of WT SENP1 were obtained as previously described for C603S SENP1 (BMRB entry19083; ref. 34 ). Backbone and side chain methyl assignments used standard through-bond NMR experiments. Stereo-specific assignments of the methyls of Val and Leu were achieved using samples produced from M9 cultures containing 20% 13 C 6 glucose and 80% unlabelled glucose as the sole carbon source [38] , [39] . All titration experiments were performed at 298 K on a Bruker Avance 600 MHz spectrometer equipped with a TXI cryoprobe. TROSY-type 1 H– 15 N HSQC spectra and constant time 1 H– 13 C HSQC for the methyl groups were collected for SENP1 and 1:1 SENP1–SUMO1 1–92 complex, without and with the addition of 2.4-fold S1-HSTV and 2.7-fold S1-GG peptides. The titration experiments for SENP1 binding to the different SUMO1 constructs, SUMO1-FL, SUMO1-GG and SUMO1 1–92 were conducted at SENP1:SUMO1 molar ratios of 1:0, 1:0.2, 1:0.4, 1:0.6, 1:0.8, 1:1.07 and 1:1.39. NMR data was processed with NMRPipe [40] , and spectra were analyzed using the programme SPARKY [41] . CSP for Fig. 3a were calculated as where Δ δ H , Δ δ N , and Δ δ C are the chemical shift differences between the free and bound states in the proton, nitrogen and carbon dimensions, respectively. 15 N relaxation measurements TROSY-type 15 N NMR relaxation experiments were performed using a [U- 15 N, 2 H]-[Ile δ1( 13 CH 3 )-Leu, Val( 13 CH 3 , 12 CD 3 )]-labelled SENP1(C603S) sample. 15 N R 1 and R 2 relaxation rates and 1 H– 15 N steady-state NOE were measured on 600 MHz Bruker spectrometer, with pulse shaping and pulsed field gradient capabilities as previously described [42] . R 1 data were recorded with relaxation delays of 100, 200 (× 2), 350, 500, 700 (× 2), 900 and 1,100 ms, and R 2 data were acquired using relaxation delays of 4.4, 8.8 (× 2), 17.6, 24.4, 35.2 (× 2), 44 and 61.6 ms. Uncertainties were estimated from duplicate points. 1 H– 15 N steady-state NOE values were determined by collecting spectra in the presence and in the absence of 3 s proton saturation, which was applied before the start of the pulse sequence. To characterize microsecond motions [27] , the decay rates of R 1ρ (2H z ′N z ), R 1ρ (2H z N z ′) and R 1ρ (2H z ′N z ′) were estimated with relaxation delays of 4, 6 (× 2), 8, 12, 16, 20, 24 (× 2), 28 and 36 ms. R 1 (2H z N z ) data was recorded using relaxation delays of 20, 30 (× 2), 40, 60, 80, 100, 120 (× 2), 140 and 170 ms. R 2 (2H x N z ), R 2 (2H z N x ) and R 2 (2H x N x ) values were converted with the equations described previously [27] . The R ex contributed from microsecond motions was calculated as where d HN =( μ 0 /4 π ) ℏ γ H γ N r HN −3 , c N = B 0 γ N Δ σ N √((1+ η N 2 /3)/3), μ 0 is the permeability of free space, ℏ is the reduced Planck’s constant, γ N and γ H are the gyromagnetic ratios of 15 N and 1 H, respectively, r HN is the averaged bond length between 1 H and 15 N nuclei. B 0 is the static magnetic field strength, Δ σ N = σ 11 −( σ 22 + σ 33 )/2, ( σ 11 , σ 22 , σ 33 ) are the principle components of the nitrogen chemical shift anisotropy tensor, η N =( σ 22 – σ 33 )/( σ 11 − σ iso ) and σ iso =( σ 11 + σ 22 + σ 33 )/3. 15 N-CPMG-relaxation dispersion experiments for free SENP1 and SUMO1 1–92 :SENP1 complex at 0.2:1 molar ratios were measured at 293 K on the Bruker Avance 600 and Ascend 700 spectrometers, using CPMG pulse sequence and phase cycling as previously described [29] . Spectra were collected as a series of two-dimensional data sets with the field strengths, ν CPMG , of 50, 100, 150, 200 (× 2), 300, 400, 500 (× 2), 600, 700, 800 and 1,000 Hz. Repeated points were used for error analysis. Each spectrum had the same CPMG duration of 40 ms and a reference spectrum was obtained using the pulse sequence without the CPMG blocks. Single-quantum 13 C-methyl relaxation dispersion experiments for free SENP1 and SUMO1 1–92 :SENP1 complex at 0.2:1 molar ratios were performed at 293 K using the same spectrometers and field strengths [30] . Data was analyzed using the MATLAB software GUARDD, with the Carver–Richards–Jones equation and Monte Carlo bootstrap method for error estimation [43] . ITC measurements ITC experiments were performed at 25 °C using a VP-ITC microcalorimeter (GE Healthcare) and with all samples buffer-matched in 50 mM Tris pH 8, 100 mM NaCl and 0 or 0.5% DMSO. SUMO1 1–92 (790 μM) was titrated into the calorimetric cell with SENP1 (C603S) at 50 μM. S1-HSTV and S1-GG peptides at 1,500 μM were titrated into the cell with SENP1 (C603S) or SENP1 (C603S) +SUMO1 1–92 (molar ratio 1:4.5), at 100 μM of SENP1 (C603S). Heats of dilution were obtained from repeating the titrations with buffer only in the calorimetric cell. Data were analyzed and fit to a single-binding site model using Origin software (Microcal). DUB-Glo assay The enzymatic reaction was performed in a total volume of 100 μl of Tris buffer (50 mM Tris, pH 8.0 and 10 mM DTT). The Z-RLRGG-Glo (DUB-Glo) substrate in the Luciferin Detection Reagent (Promega) was mixed with WT SENP1 (final concentration: 100 nM) or WT SENP1–SUMO1 1–92 complex (1:75 molar ratio) in a white 96-well plate at 0–130 μM final concentration. The molar ratio used for the complex was based on optimal concentrations that ensured SENP1 saturation (>70%) without aggregation. Similarly, the USP5:Ubi (1:1,500) was subjected to the same experimental procedure using 100 nM USP5. Triplicate experiments were carried out for error estimation. Luminescence was recorded at 25 °C and 30 min after the addition of the enzyme according to the recommendation from Promega. The correlation between the measured RLU (relative light unit) of fully cleaved DUB-Glo substrate and the corresponding known substrate concentration was used to convert RLU to molar concentration. The data was analyzed using GraphPad Prism software and was fit to the Michaelis–Menten kinetics model with nonlinear regression. How to cite this article : Chen, C.-H. et al . Conformational flexibility and changes underlying activation of the SUMO-specific protease SENP1 by remote substrate binding. Nat. Commun. 5:4968 doi: 10.1038/ncomms5968 (2014). Accession codes : Chemical shift assignments for wild-type SENP1 catalytic domain have been deposited in the Biological Magnetic Resonance Bank under the accession code 19,885 .